The microbiome extends to subepidermal compartments of normal skin Commensal microbes on the skin surface influence the behaviour of cells below the epidermis. We hypothesized that bacteria or their products exist below the surface epithelium and thus permit physical interaction between microbes and dermal cells. Here to test this hypothesis, we employed multiple independent detection techniques for bacteria including quantitative PCR, Gram staining, immunofluorescence and in situ hybridization. Bacteria were consistently detectable within the dermis and dermal adipose of normal human skin. Sequencing of DNA from dermis and dermal adipose tissue identified bacterial 16S ribosomal RNA reflective of a diverse and partially distinct microbial community in each skin compartment. These results show the microbiota extends within the dermis, therefore, enabling physical contact between bacteria and various cells below the basement membrane. These observations show that normal commensal bacterial communities directly communicate with the host in a tissue previously thought to be sterile. The epithelial surfaces of the human body engage in mutualistic relationships with vast and complex microbial populations. The resident microbiota of the skin is particularly diverse because human skin provides several unique environmental niches that differ in humidity, temperature, pH, antimicrobial peptide (AMP) composition and lipid content [1] , [2] . Previous analyses of the surface microbial composition at different cutaneous sites has established that the capacity to detect microbes is dependent on the specific characteristics of the site sampled [3] , [4] and remains relatively stable over time within an individual despite the dramatic changes that often occur in the outside environment [5] . These observations suggest the skin may communicate with microbes at the surface to actively regulate, which organisms populate it. Further evidence that communication takes place between surface microbes and deeper host cells comes from data showing that components of the skin commensal microbial community affect the development of the immune system and the physical characteristics of the epidermal barrier [6] , [7] , [8] , [9] , [10] . Thus, although it is becoming increasingly accepted that a dynamic interaction takes place between the surface bacteria and the host, it is currently unclear how this can take place if the microbial community resides only on top of a physical barrier devoid of live cells. Below the surface of the stratum corneum there are many cells that are well equipped to detect and respond to microbes. The deep epidermis and dermis is composed of many different specialized cell types that each express unique repertoires of functional pattern-recognition receptors, and these receptors actively respond when exposed to components of microbes in vitro [11] , [12] , [13] , [14] . The influence of surface microbes on cutaneous immune function led us to question the assumption that the skin maintains a complete barrier to bacterial entry, and to hypothesize that that some microbes or their products may penetrate below the stratum corneum and perhaps below the basement membrane of the epidermis. In this study, we show that diverse elements of the skin microbiome are present in subcutaneous regions of normal human skin and are, therefore, directly positioned to influence the host behaviour. Bacterial DNA is detectable deep in normal human skin To determine the relative abundance of microbial DNA below the superficial barrier of the skin stratum corneum, subject skin was subjected to surgical scrubbing and sterile swabbing before biopsy for DNA analysis. Quantitative measurements of 16S ribosomal RNA (rRNA) gene abundance were done by real-time quantitative PCR (qPCR) with universal primers in sequential horizontal sections of normal human skin ( Fig. 1a and Supplementary Fig. S1 ). Multiple samples of facial and palm skin from different donors were evaluated, with palm skin chosen because of the absence of hair follicles and a thick stratum corneum. Quantification of the 16S rRNA gene was influenced by neither the presence of human genomic DNA nor optimal cutting temperature (OCT) tissue embedding compound ( Supplementary Fig. S2a,b ). In addition, no bacterial DNA contamination was detectable in the reagents used for these experiments ( Supplementary Fig. S2c ). Our procedures detect the existence of DNA encoding for bacterial 16S rRNA genes at various depths in subcutaneous tissues. Notably, 16S rRNA genes were detected beneath the maximal depth of follicles in facial skin (3.0 mm) and below the eccrine glands that extended 1.5 mm below the surface in palm skin ( Supplementary Fig. S3 ). PCR amplification was negative of control samples from surrounding OCT embedding compound or in reagents used to process the tissue sections. 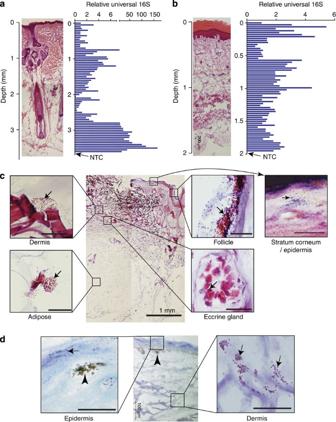Figure 1: Bacterial components are detectable deep in normal human skin. (a,b) Total DNA was extracted from sequential 30 or 50 μm horizontal sections of 6-mm punch biopsies of human facial (a) or palm skin (b). 16S rRNA gene was quantified with real-time qPCR using universal 16S rRNA primers. Relative abundance of 16S rRNA gene was calculated by the ΔCt method. Haematoxylin and eosin staining of each skin biopsy is shown in the same scale as theyaxis of the graph. Arrow indicates data from the DNA sample prepared from a non-tissue control (NTC) that represents a section of OCT embedding compound devoid of tissue and processed with all reagents used for amplification of tissue sections. SeeSupplementary Fig. S1for additional biopsy data from different donors. (c) Gram staining of frozen sections from normal human facial skin. SeeSupplementary Fig. S4for additional biopsy data from different donors. (d) To examine if bacteria are associated with CD11c+cells, normal human facial skin was Gram stained (purple/red: arrow), and then stained with anti-CD11c monoclonal IgG (brown: arrow head). Scale bar, 20 μm. Figure 1: Bacterial components are detectable deep in normal human skin. ( a , b ) Total DNA was extracted from sequential 30 or 50 μm horizontal sections of 6-mm punch biopsies of human facial ( a ) or palm skin ( b ). 16S rRNA gene was quantified with real-time qPCR using universal 16S rRNA primers. Relative abundance of 16S rRNA gene was calculated by the ΔCt method. Haematoxylin and eosin staining of each skin biopsy is shown in the same scale as the y axis of the graph. Arrow indicates data from the DNA sample prepared from a non-tissue control (NTC) that represents a section of OCT embedding compound devoid of tissue and processed with all reagents used for amplification of tissue sections. See Supplementary Fig. S1 for additional biopsy data from different donors. ( c ) Gram staining of frozen sections from normal human facial skin. See Supplementary Fig. S4 for additional biopsy data from different donors. ( d ) To examine if bacteria are associated with CD11c + cells, normal human facial skin was Gram stained (purple/red: arrow), and then stained with anti-CD11c monoclonal IgG (brown: arrow head). Scale bar, 20 μm. Full size image Detection of microbial components below the epidermis We could not completely rule out the possibility that bacteria detected by horizontal sectioning and real-time qPCR was from the presence of appendageal structures known to harbour bacteria. Therefore, to further assess the location of bacteria in the dermis, we next sought to identify bacteria in the dermis of normal human facial skin by independent staining techniques. Gram staining visualizes structures that appear to be bacteria in locations where they are expected, such as the stratum corneum, hair follicles and eccrine glands ( Fig. 1c and Supplementary Fig. S4 ). However, similar structures that appear to be bacteria are also detectable by Gram staining in both reticular dermis and dermal adipose. These regions are not physically connected with the surface. To determine if the presence of bacteria in the dermis was associated with phagocytic cells that may have engulfed bacteria in transit, sections were also counter-stained with anti-CD11c antibody. Most bacteria visualized by Gram staining are distributed throughout the dermis independently of CD11c + immunoreactivity ( Fig. 1d ), thus suggesting they are not in classical phagocytic immune cells. Specific immunostaining was performed next for Staphylococcus epidermidis ( S. epidermidis ), an abundant species that is cultivable from normal human skin surface, and Pseudomonas spp. , a genus that has been reported by 16S rRNA gene sequencing approaches in one study performed on skin biopsies as being present in normal human skin [15] . S. epidermidis is routinely detected below the epidermal basement membrane ( Fig. 2a—d and Supplementary Fig. S5a–f ). Pseudomonas spp. are also readily detected in the dermis, and are present outside of appendageal structures identified by keratin 14 staining ( Fig. 2e–h ). In addition to DNA for 16S rRNA, other bacterial products can also be detected in the dermis by immunostaining approaches with anti-lipopolysaccharide, and is co-localized with collagen-I, the most abundant collagen in the dermis ( Fig. 2i ). Similarly to the Gram staining data ( Fig. 1d ), immunostaining with anti-CD11c fails to detect these bacterial products within immune cells ( Fig. 2i ). No immunoreactivity is detected by isotype control IgGs for each antigen-specific antibody (Fig. 5c,d,f,h,j). All immunostaining is reproducible in multiple skin biopsies from different donors ( Supplementary Fig. S5a–l ). Bacterial 16S rRNA is also detectable in dermal adipose tissue of normal facial skin by in situ hybridization with an oligonucleotide probe EUB338 ( Fig. 2k and Supplementary Fig. S5o ). This probe also detects 16S rRNA in the eccrine gland that connects to the surface ( Supplementary Fig S5m,q ), a site expected to have some bacteria. No signal was detectable with a control nonsense probe (nonEUB338) ( Fig. 2l and Supplementary Fig. S5n,p,r ). 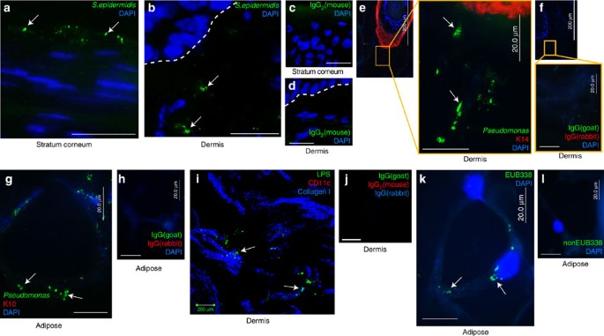Figure 2: Detection of microbes in normal human skin by immunostaining andin situhybridization. (a–d) Normal human facial skin was stained with anti-S. epidermidismonoclonal IgG (a,b) or isotype IgG (c,d). The broken line depicts the basement membrane of the epidermis. (e–h) Normal human facial skin was stained with anti-Pseudomonas spp. (green) and anti-keratin 14 (K14) (red) (e,g), or isotype control IgGs (f,h). (i,j) Lipopolysaccharide (LPS) was detectable in the reticular dermis of facial skin sections stained with anti-LPS (green) and was associated with collagen fibres detected by anti-collagen-I staining (blue). Phagocytic cells stained with anti-CD11c IgG (red) were undetectable (i). Control IgGs for LPS, collagen-I and CD11c were negative in adjacent sections (j). (k,l) Bacterial 16S rRNA was detectable in normal human facial skin sections hybridized with an Alexa Fluor488-labelled EUB338 probe. Specific hybridization was detected in dermal adipose tissue (k). No signal was seen in adjacent sections hybridized with a nonsense control probe (nonEUB338) (l). SeeSupplementary Fig. S5for additional biopsy data from different donors. Scale bar, 20 μm, if not indicated. DAPI, 4′,6-diamidino-2-phenylindole. Figure 2: Detection of microbes in normal human skin by immunostaining and in situ hybridization. ( a – d ) Normal human facial skin was stained with anti- S. epidermidis monoclonal IgG ( a , b ) or isotype IgG ( c , d ). The broken line depicts the basement membrane of the epidermis. ( e – h ) Normal human facial skin was stained with anti- Pseudomonas spp . (green) and anti-keratin 14 (K14) (red) ( e , g ), or isotype control IgGs ( f , h ). ( i , j ) Lipopolysaccharide (LPS) was detectable in the reticular dermis of facial skin sections stained with anti-LPS (green) and was associated with collagen fibres detected by anti-collagen-I staining (blue). Phagocytic cells stained with anti-CD11c IgG (red) were undetectable ( i ). Control IgGs for LPS, collagen-I and CD11c were negative in adjacent sections ( j ). ( k , l ) Bacterial 16S rRNA was detectable in normal human facial skin sections hybridized with an Alexa Fluor488-labelled EUB338 probe. Specific hybridization was detected in dermal adipose tissue ( k ). No signal was seen in adjacent sections hybridized with a nonsense control probe (nonEUB338) ( l ). See Supplementary Fig. S5 for additional biopsy data from different donors. Scale bar, 20 μm, if not indicated. DAPI, 4′,6-diamidino-2-phenylindole. Full size image The subcutaneous microbiome is diverse The detection of bacterial antigens and 16S rRNA in the dermis by multiple histological approaches supports initial qPCR results that suggest bacterial products are present deep in the skin. To further confirm the identity of PCR products amplified by universal 16S rRNA primers, and begin to investigate the diversity of microbial DNA in regions of the dermis devoid of appendageal structures, a laser-capture microdissection (LCM) technique was employed ( Supplementary Fig. S6 ) in conjunction with 16S rRNA gene pyrosequencing. 16S rRNA gene fragments were amplified from distinct tissue compartments including the follicle, epidermis, dermis, adipose tissue and a region of OCT embedding compound as a non-tissue control. Amplification of 16S rRNA gene fragments by barcoded primers was confirmed by gel electrophoresis before 454-pyrosequencing. No amplicons were generated from NTC samples. Each sample containing skin tissue yields >10,000 sequences, whereas samples generate only 20 reads. Furthermore, 14 of these negligible number of reads from NTC samples correspond with Proteobacteria sequences, in which two sequences were assigned as Pseudomonadales (order), a finding consistent with previous reports of contaminating bacterial DNA from negative extraction controls [16] . Rarefaction analyses shows that the number of reads obtained by pyrosequencing are adequate to obtain nearly saturating numbers of species in the samples ( Supplementary Fig. S7 ), whereas only nine OTUs are assigned in the reads of NTC samples. The microbial DNA in all skin compartments consists primarily of members of the phylum Proteobacteria with proportionally less representation of other phyla, such as Actinobacteria, Firmicutes and Bacteroidetes ( Fig. 3a ). Taxonomic classification at the order level is also shown ( Supplementary Table S1 ). 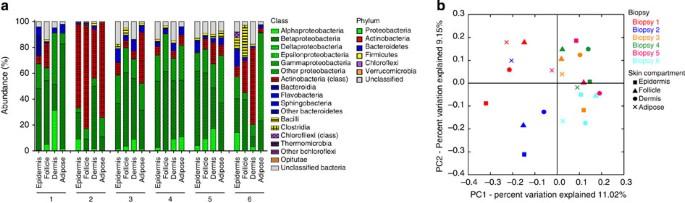Figure 3: The subcutaneous microbiome is diverse. (a) The profile of the subcutaneous microbiome at the class level derived from pyrosequencing analysis of DNA encoding the 16 S rRNA gene. Relative abundance of bacterial classes associated with each skin compartment is shown for each skin biopsy. (b) Principal coordinate plot analysis displaying similarity of composition of bacterial 16S rRNA gene sequences contained in each cutaneous compartment. Each symbol corresponds to the sample of epidermis(), follicle(), dermis() and adipose tissue (×). The biopsy number is shown in different colour and identical to the data inFig. 3a. Figure 3: The subcutaneous microbiome is diverse. ( a ) The profile of the subcutaneous microbiome at the class level derived from pyrosequencing analysis of DNA encoding the 16 S rRNA gene. Relative abundance of bacterial classes associated with each skin compartment is shown for each skin biopsy. ( b ) Principal coordinate plot analysis displaying similarity of composition of bacterial 16S rRNA gene sequences contained in each cutaneous compartment. Each symbol corresponds to the sample of epidermis( ), follicle( ), dermis( ) and adipose tissue (×). The biopsy number is shown in different colour and identical to the data in Fig. 3a . Full size image To further compare taxonomic profiles in each skin compartment, quantitative insights into microbial ecology (QIIME) based principal coordinate analysis was performed ( Fig. 3b ). Taxonomic composition is highly divergent between skin samples from individual donors. In addition, the taxonomic composition in each cutaneous compartment does not completely overlap even within the same specimen, suggesting each skin compartment may harbour somewhat unique microbe communities. Bacterial DNA is detectable in subepidermal compartments Although pyrosequencing is an ideal tool for exploring the vast majority of rare and often uncultivable microbes in complex microbial communities, the approach is less well suited for an absolute quantification of abundance of specific microbe within the community. To address this technical limitation, real-time qPCR was performed on LCM samples using universal 16S rRNA primers and genus- or species-specific primer/probes. The lowest detection limit of real-time qPCR is 1-10 colony-forming unit (CFU) equivalent for universal 16S rRNA gene, P. acnes and S. epidermidis , and 10-100 CFU equivalent for Pseudomonas spp . As hair follicles and epidermal LCM sections were from regions in contact with the surface, and thus expected to have abundant bacterial DNA, the results using universal 16S rRNA primers on these regions serve as a positive control. In addition to the positive results from regions known to have abundant bacteria, a consistent universal 16S rRNA gene product is also detected by real-time qPCR in LCM-isolated sections from dermal and adipose tissue ( Fig. 4a ), regions previously thought to be devoid of microbes. To rule out that the qPCR signals from these regions are due to contamination of these samples, DNA extraction and amplifications were simultaneously performed on the buffers and reagents alone, on adjacent LCM specimens isolated from regions on the slide that did not contain skin ( Supplementary Fig. S6 , NTC), and on skeletal muscle biopsies prepared with the same reagents used to isolate DNA from dermal and adipose LCM. These negative control samples do not yield a positive signal ( Fig. 4a ). 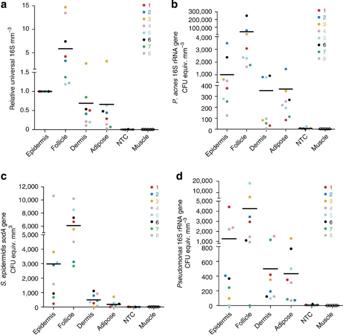Figure 4: Measurement of abundance of bacterial DNAs in subepidermal compartments. (a–c) Abundance of universal bacterial 16S rRNA gene (a),P. acnes-specific 16S rRNA gene (b),S. epidermidis sodAgene (c), orPseudomonas-specific 16S rRNA gene (d) was measured by real-time qPCR. Relative abundance of DNA for 16S rRNA gene was calculated with a ΔCt method.P. acnesandS. epidermidiswere quantified by comparison with known CFUs of these organisms.Pseudomonasspecies was quantified by comparison with known CFUs ofP. aeruginosa. Skin compartments including epidermis and stratum corneum, follicle, dermis and subcutaneous adipose tissue was excised by LCM. Non-tissue control (NTC) processed from embedding material adjacent to the tissue sample, and sterile skeletal muscle biopsy tissue, are also shown as negative controls to detect contamination. Each point represents a separate individual skin biopsy. The biopsy number is shown in different colour and identical to the data inFig. 3a. The skeletal muscle specimens shown were obtained from five different donors. Figure 4: Measurement of abundance of bacterial DNAs in subepidermal compartments. ( a – c ) Abundance of universal bacterial 16S rRNA gene ( a ), P. acnes -specific 16S rRNA gene ( b ), S. epidermidis sodA gene ( c ), or Pseudomonas -specific 16S rRNA gene ( d ) was measured by real-time qPCR. Relative abundance of DNA for 16S rRNA gene was calculated with a ΔCt method. P. acnes and S. epidermidis were quantified by comparison with known CFUs of these organisms. Pseudomonas species was quantified by comparison with known CFUs of P. aeruginosa . Skin compartments including epidermis and stratum corneum, follicle, dermis and subcutaneous adipose tissue was excised by LCM. Non-tissue control (NTC) processed from embedding material adjacent to the tissue sample, and sterile skeletal muscle biopsy tissue, are also shown as negative controls to detect contamination. Each point represents a separate individual skin biopsy. The biopsy number is shown in different colour and identical to the data in Fig. 3a . The skeletal muscle specimens shown were obtained from five different donors. Full size image Bacteria-specific primers/probes were next designed to evaluate the abundance of candidate genes from Propionibacterium acnes ( P. acnes ), S. epidermidis and Pseudomonas spp. . Use of gene-specific primers/probes permits abundance to be quantified by comparison to known standard amounts of these organisms. DNA encoding P. acnes -specific 16S rRNA, S. epidermidis sodA and Pseudomonas 16S rRNA is detectable in most of DNA samples extracted from each skin compartment tested ( Fig. 4b–d , respectively). Cross-contamination of bacteria between compartments, or from the processing environment, is negligible as detected by simultaneous qPCR analysis of OCT embedding material adjacent to each tissue, or human muscle biopsies. Direct sequencing of qPCR products confirmed that the PCR amplicons were consistent with the predicted targeted gene sequences ( Supplementary Tables S2-4 ). This study shows evidence of a previously unknown physical interaction that routinely occurs between commensal bacteria and dermal cells. This interaction was particularly surprising in the deep dermal stroma and superficial adipose tissue, areas that were traditionally assumed to be devoid of a microbial community in the absence of skin injury. In particular, bacterial products including DNA encoding for 16S rRNA genes, bacteria-specific antigens and bacterial rRNA were ubiquitously detected throughout subcutaneous regions of normal human skin. These observations provide the first evidence of a physical interaction between commensal bacteria and living dermal cells deep in normal skin. This study does not prove that live bacteria colonize or inhabit the dermis, as the approaches used here are unable to distinguish between viable and dead cells. Microorganisms do not have to be alive to exert influence on the host immune system. Bacterial components or products, including lipoteichoic acid (LTA), commensal microbial DNA, ATP and polysaccharide A, can all exert effects on host cells [6] , [7] , [8] , [9] , [17] , [18] , [19] . It is, however, possible that some microbes do survive below the epithelial barrier but cannot be successfully cultured by current techniques. Supporting this was the detection of 16S rRNA with in situ hybridization in superficial adipose tissue. Bacterial RNA is rapidly degraded after cell death [20] , thus it would not be expected to obtain strong 16S rRNA hybridization signals from dead cells. The microbiota residing in superficial layers or appendage structures might be translocated into the subepidermal compartments by phagocytic cells. However, most dermal bacteria existed independently of CD11c, and thus the route of entry remains to be determined. Notably, pyrosequencing revealed that the diversity of bacterial 16S rRNA genes in each skin compartment within the same specimen was not identical to the surface composition. Further studies are necessary to understand the mechanisms by which the skin permits commensal bacteria to enter across the epidermal barrier. High interpersonal variability was observed in the current study of subcutaneous microbial communities. This variability requires further in depth study, but is similar to prior observations of the surface skin microbiome [5] . In past reports, Propionibacterium and Staphylococcus spp. were predominantly detected on the surface of sebaceous sites when collected by superficial sampling methods, whereas Proteobacteria were relatively less frequent [3] . In this study, we observed high proportions of Proteobacteria, including Burkholderiales and Pseudomonadales, and Actinobacteria, but a relatively lower proportion of Firmicutes in subepidermal compartments of facial skin. Furthermore, in prior reports, proteobacteria, including Pseudomonas spp. and Janthinobacteria spp . or β-proteobacteria class, were relatively predominant in the superficial swab samples from forearm skin [3] , [15] , [21] . We cannot conclude here why our observation differ from previous reports. In particular, other studies of the superficial skin microbiome have failed to detect a predominant proportion of Pseudomonas species [4] , [5] , and it remains an unresolved question as to the inconsistencies between prior studies using similar techniques. However, it is important to reiterate that our results cannot be compared directly to the previous reports of resident microflora on the skin surface as we washed the skin with a disinfectant cleanser before skin biopsy. Cleaning the stratum corneum and potentially altering the skin barrier is likely an important factor affecting microbiome analysis. The validity of our data from LCM was supported by qPCR results, and further confirmed by direct sequencing of qPCR products from these reactions. Also, data were consistent with the expected results from sites with known bacterial populations such as a high abundance of S. epidermidis detected in the epidermis and an increased abundance of P. acnes in the anaerobic and lipid-rich hair follicle. Future analysis of the dermal microbial communities can provide a more accurate taxonomic profile by using a combination of 454-pyrosequencing and paired-end Illumina shotgun sequencing [22] . Therefore, although precise identification of the dermal bacteria is not shown here, the data strongly support the conclusion that a diverse microbial community is present in the dermis. Our study also suggests individuals may have unique subsets of the total microbial population in each cutaneous compartment. This observation permits the novel hypothesis that the human skin actively regulates bacterial entry or penetration into dermis. Epidermal physical barriers or AMPs may be key regulators to maintain dermal microbiome homoeostasis. In addition, bacterial mechanisms to escape from the host immune response may also contribute to the development of the dermal microbiome. For example, a wide variety of Gram-negative bacteria produce N -homoserine lactone [23] , which selectively impairs the regulation of toll-like receptor-dependent nuclear factor kappa-light-chain-enhancer of activated B cell functions [24] . Bacteria in biofilms are known to evade host immune responses and to be much less susceptible to killing by AMPs [25] , [26] , [27] . Indeed, multiple independent staining techniques detected aggregated bacteria in the subepidermal compartments. These mechanisms may facilitate bacterial entry and/or persistence in the dermis. Finding bacteria in the dermis is surprising but it helps explain multiple lines of recent evidence that show that cells below the physical barrier of the skin’s stratum corneum will respond to factors produced by commensal microbes. For example, a unique lipoteichoic acid produced by S. epidermidis inhibits cytokine production from basal keratinocytes induced by RNA released from damaged cells [7] . A small component secreted from S. epidermidis increases expression of β-defensins in murine skin and human keratinocytes [8] . S. epidermidis -conditioned media strongly enhances AMP production induced by S. aureus in keratinocytes [9] . Middle- or long-chain-free fatty acids, mostly produced via hydrolysing sebum triacylglycerides by bacterial lipases, enhance production of β-defensins in sebocytes [28] . More recently, it has been demonstrated that skin commensal bacteria enhanced cutaneous T-cell functions via activation of interleukin-1 signaling [10] . Indeed, mono-colonization of germ-free mouse skin by S. epidermidis rescued protection against pathogen infection in comparison to germ-free skin. Several lines of evidence have also shown that disruption of normal interactions between the host and the skin microbiome is associated with skin disorders [29] , [30] . Our observations here that the bacterial community can extend to deep within the skin shows how the microbiome may exert such effects on the host. In the future, further studies are required to understand how the dermal microbiome influences the function of dermal cells. Germ-free mice will be a strong tool to evaluate the roles of the dermal microbiome [7] , [10] . In addition, the significance of our current observations may provide a better understanding of how the skin microbial ecology can trigger disease. Indeed, atopic dermatitis, psoriasis and rosacea have all been associated with altered skin barrier function [31] . Alterations in barrier function may result in dysbiosis of the subcutaneous microbiome and contribute to the pathogenesis of diseases not considered to be primarily of infectious aetiology. It will be of interest to investigate how altered skin barrier function impacts the subcutaneous microbiome and how this contributes to disease. Thus, this study expands our understanding of the complexity of symbiotic interactions between our microbial community and human health and provides the basis for an entirely new approach to understanding skin disease. Preparation of normal human skin All experiments involving human subjects were carried out according to the Institutional Review Board protocols approved by the UC San Diego (Project#071032). Normal human facial and palm skin was aseptically obtained from excess healthy tissue removed during sterile surgical procedures for excision of non-melanoma skin cancers. The donors included five males and three females in a range of 54–67-years-old for facial skin and two males and one female in a range of 53–69-years-old for palm skin. Skin was disinfected before surgery. To avoid contamination of surface bacteria not removed by surgical scrub of the skin before excision, and to further isolate samples from potential contamination, a 6-mm sterile biopsy was excised from the centre of the excess normal skin samples immediately after surgery. This sample was removed by cutting from the dermis to the epidermis on a sterile surgical field to avoid passive transfer of surface microbes during the excision process. Sequential 30 or 50 μm horizontal sections of frozen skin were then prepared from the 6-mm biopsy by cutting from the dermis side towards the epidermis with a cryostat blade that was cleaned with alcohol after obtaining each section. Staining of bacteria To visualize bacteria, Gram staining of normal facial human skin was performed with Gram staining kit for tissue (Sigma, St Louis, MO, USA). To examine if subcutaneous microbiome is associated with CD11c + cells, normal human facial skin was fixed with 3.7% formalin, stained by Gram staining, and then stained with anti-CD11c monoclonal IgG (Santa Cruz Biotechnology, Inc., Santa Cruz, CA). The immunoreactivity for CD11c was visualized with anti-mouse IgG-HRP conjugate, followed by DAB. To detect S. epidermidis , cryostat sections of normal human facial skin were fixed, blocked, and incubated with MEP_L_cop3anti-S. epidermidis monoclonal IgG (5 μg ml −1 ) (Santa Cruz Biotechnology, Inc.) for 1 h, followed by anti-mouse IgG-Alexa 488 conjugate (2 μg ml −1 ) (Invitrogen) for 30 min. To detect Pseudomonas spp ., cryostat sections of normal human facial skin were fixed and incubated with Endogenous Biotin-Blocking Kit (Invitrogen, Carlsbad, CA, USA). After blocking, the sections were incubated with biotinylated rabbit anti-Pseudomonas species IgG (5 μg ml −1 ) (Thermo Scientific, Waltham, MA, USA) for 1 h, followed by streptavidin-Alexa 488 conjugate (2 μg ml −1 ) (Invitrogen) for 30 min. Biotinylated normal rabbit IgG was used as a negative control for the detection. To visualize epithelia, the sections were stained with Goat-anti-K14 IgG (1 μg ml −1 ) (Santa Cruz Biotechnology), followed by rabbit anti-goat IgG-Alexa 568 (1 μg ml −1 ) (Invitrogen). To examine localization of lipopolysaccharide in the reticular dermis, normal human facial skin was stained with goat anti-LPS polyclonal IgG (Novus, Litteton, CO, USA), mouse anti-CD11c monoclonal IgG and rabbit anti-collagen type-I (Santa Cruz Biotechnology), followed by Donkey anti-Goat IgG-Alexa 488, anti-mouse Alexa 594 and anti-rabbit Alexa 350 (Invitrogen). The confocal image was obtained using Zeiss LCM510 (Carl Zeiss, Germany). For fluorescence in situ hybridization, oligonucleotide probes (EUB338: 5′-GCTGCCTCCCGTAGGAGT-3′) targeting 16 S rRNA of most bacteria was labelled with Alexa flour 488 (Invitrogen) [32] . Cryostat sections of normal human facial skin were immediately fixed with RNase-free 4% formaldehyde and permeabilized, followed by dehydration with 50, 75, 100% ethanol. The sections were hybridized with EUB338 (5 ng ml −1 ) in in situ hybridization buffer (Enzo Life Science, Farmingdale, NY, USA). Alexa flour 488-labelled non-EUB338, reverse complement of EUB338, was used for a control staining. The excess probe and nonspecific binding were washed with 2 × saline-sodium citrate containing 16% formaldehyde at 60° C. Laser-capture microdissection Twenty micrometre cryostat sections of normal human facial skin were mounted on a nucleic acid-free membrane slide (MMI, Haslett, MI, USA), stained with methylene blue to visualize appendageal structures, and immediately dehydrated with Arcturus dehydration components (Applied Biosystems, Foster City, CA, USA). Epidermis including stratum corneum, follicle, reticular dermis or subcutaneous adipose tissue was excised with a microdissection system (MMI). Subcutaneous compartments were carefully cropped to avoid appendageal structures when not intentionally included. A NTC was excised from a region of the OCT section on the film slide downstream from the blade after passing through the tissue sample. Human muscle tissue biopsies generously provided by Dr Richard Lieber, UCSD Institutional Review Board #071702, were used as an additional control of sterile tissue. These sections were processed together with the sections containing skin to detect potential contaminants introduced by the sectioning process, instruments, DNA extraction solutions and PCR amplification reagents. The excised area was determined to normalize the data into tissue volume (20 μm thickness × area μm 2 ). DNA extraction Skin sections or microdissected samples were lysed with proteinase K, followed by purified achromopeptidase (Wako, Osaka, Japan) to ensure bacterial cell lysis. Total genomic DNA was purified with QIAamp DNA mini kit (Qiagen) or from microdissected skin compartment with NucleoSpin (Macherey-Nagel, Duren, Germany). Quantification of bacteria by real-time qPCR Relative abundance of the DNA present encoding bacterial 16S rRNA was evaluated with real-time qPCR with the universal 16S rRNA primer set, 1048-F and 1175-R ( Supplementary Table S5 ). The universal primer set covers 79% of Proteobacteria, 85% of Actinobacteria, 72% of Firmicutes and 61% of Bacteroidetes [33] . Abundance of P. acnes or S. epidermidis , the dominant cultivable species in human skin, was determined with the gene-specific primers/probe targeting the P. acnes -specific sequence of 16S rRNA gene and primers targeting S. epidermidis -specific sequence of sodA ( Supplementary Table S5 ) [34] , [35] . Abundance of Pseudomonas spp. was determined with the genus-specific primer/ probe targeting Pseudomonas 16S rRNA ( Supplementary Table S5 ) [36] , [37] . PCR was performed with Power SYBR Green Master mix to determine total DNA abundance for the 16S rRNA gene and S. epidermidis sodA DNA, TaqMan Universal Master mix (Applied Biosystems) or Maxima Probe/ROX qPCR Master Mix (Thermo Scientific) to determine P. acnes 16S rRNA and Pseudomonas -genus specific 16S rRNA gene, respectively. Thermal cycling conditions used were as follows; for total 16S rRNA DNA and S. epidermidis sodA DNA, 50 °C for 2 min and 95 °C for 10 min, 40 cycles of 95 °C for 15 s, 60 °C for 1 min, followed by dissociation stage; for P. acnes and Pseudomonas spp. 16S rRNA DNA, 50 °C for 2 min and 95 °C for 10 min, followed by 50 cycles of 95 °C for 15 s 60 °C for 1 min. Because of a lack of standard bacteria that can be used as an external control of absolute quantification for universal 16S rRNA gene abundance, the relative abundance of this DNA in different skin sections or LCM samples was calculated with a ΔCt method and then normalized to the tissue volume excised. To determine absolute abundance of specific bacterial species, a standard curve was generated with genomic DNA extracted from standards derived from known amounts of CFU of P. acnes (ATCC6919), S. epidermidis (ATCC12228) and P. aeruginosa (ATCC14213), and then the quantity was normalized to the tissue volume excised. The specificity of all primer pairs was confirmed by melting curve analysis and DNA electrophoresis of PCR amplicons. To further evaluate the specificity species- or genus- specific primers/probe, each qPCR amplicon was cloned into pGEM-T plasmid (Promega, Madison, WI, USA) and the insert was sequenced. Microbiome profiling by pyrosequencing Bacterial tag-encoded FLX amplicon pyrosequencing (bTEFAP) was performed at the Research and Testing Laboratory (Lubbock, TX, USA). Initial generation of the sequencing library utilized Gray28F and Gray519R primer set ( Supplementary Table S5 ) lacking tag sequences to amplify variable regions V1-V3 of 16S rRNA gene with enhanced specificity in samples containing abundant mammalian DNA. The second PCR was performed using designed unique fusion primers with different tag sequences ( Supplementary Table S6 ). Thermal cycling conditions used were as follows; 95 °C for 5 min, then 15 cycles (1st PCR) or 20 cycles (2nd PCR) of 94 °C for 30 s, 54 °C for 40 s, 72 °C for 1 min, followed by one cycle of 72 °C for 10 min. PCR products were then pooled equimolar and each pool was cleaned with Diffinity RapidTip (Diffinity Genomics, West Henrietta, NY, USA), and size selected using Agencourt AMPure XP (BeckmanCoulter, Indianapolis, IN, USA) following Roche 454 protocols (454 Life Sciences, Branford, CT, USA). Size selected pools were then quantified and 150 ng of DNA were hybridized to Dynabeads M-270 (Life Technologies) to create single-stranded DNA following Roche 454 protocols (454 Life Sciences). Single-stranded DNA was diluted and used in emPCR reactions, which were performed and subsequently enriched as described in the manufacturer’s protocols (454 Life Sciences). bTEFAP analyses were performed with a 454 FLX instrument (Roche, Basel, Switzerland) as described previously [38] , [39] . The QIIME software package (version 1.5.0) [40] was used for quality control of the raw sequence reads using the split_library.py script and the following criteria: (1) no ambiguity base allowed and no mismatches allowed in the primer sequence; (2) minimum and maximum length of 200 bp and 1,000 bp; (3) an minimum quality score of 25. Sequences were binned based on sample-specific barcode sequences and trimmed with removal of the barcode and primer sequences. High quality sequence reads were first de-replicated using 97% similarity and the potential chimeric sequences were detected using the UCLUST software package [41] , [42] . Chimeric sequences were removed before taxonomic assignments. To obtain taxonomic identities of clustered operational taxonomic units (OTUs) by UCLUST, the RDP database and classifier [43] was used to assign taxonomy at the confidence threshold >80%. OTU sequences that did not return any confident hit with RDP classification algorithrm were labelled as ‘no match’. Finally, the taxonomic composition for each sample is summarized in bar chart at the taxonomic levels of class. To compare taxonomic profiles in different skin compartments from each skin biopsy, alpha and beta diversity, principal coordinate analysis and rarefaction analyses were carried out in the QIIME pipeline [40] . Accession codes: Sequence data have been deposited in the DDBJ Sequence Read Archive under accession code PRJDB716 . How to cite this article: Teruaki Nakatsuji et al. The microbiome extends to subepidermal compartments of normal skin. Nat. Commun. 4:1431 doi: 10.1038/ncomms2441 (2013).